Aerodynamic performance of the feathered dinosaurMicroraptorand the evolution of feathered flight Understanding the aerodynamic performance of feathered, non-avialan dinosaurs is critical to reconstructing the evolution of bird flight. Here we show that the Early Cretaceous five-winged paravian Microraptor is most stable when gliding at high-lift coefficients (low lift/drag ratios). Wind tunnel experiments and flight simulations show that sustaining a high-lift coefficient at the expense of high drag would have been the most efficient strategy for Microraptor when gliding from, and between, low elevations. Analyses also demonstrate that anatomically plausible changes in wing configuration and leg position would have made little difference to aerodynamic performance. Significant to the evolution of flight, we show that Microraptor did not require a sophisticated, ‘modern’ wing morphology to undertake effective glides. This is congruent with the fossil record and also with the hypothesis that symmetric ‘flight’ feathers first evolved in dinosaurs for non-aerodynamic functions, later being adapted to form lifting surfaces. Ever increasing numbers of feathered non-avialan dinosaurs have revolutionized our understanding of bird-flight origins [1] , [2] , [3] . The fossil record shows that a variety of paravians closely related to, but outside, the avialan clade possessed feathered flight surfaces; the best represented of these is the Early Cretaceous dromaeosaurid Microraptor [4] . This dinosaur possessed elongated arm, leg and tail feathers [4] , an anatomical configuration that resurrected an older idea that paravian flight passed through a four-winged (‘tetrapteryx’) phase. However, even in light of new fossil discoveries, the evolution of bird flight remains one of the greatest debates in biology and palaeontology; for more than 160 years, evolutionary scenarios have been developed to explain the evolution of this major adaptation [1] . Flapping flight using asymmetric feathers (which is a prerequisite shape for feathers to be aerodynamically stable when orientated other than parallel to the airflow) has long been thought to distinguish birds from the other vertebrate fliers, bats and pterosaurs [2] . Exceptional Mesozoic-aged ( ca. 140–66 Myo) fossils have closed the anatomical gap between non-avialan dinosaurs and birds (Avialae) [3] and have demonstrated that feathers (including asymmetric flight feathers) are not uniquely avialan adaptations [4] , [5] . Within the region of the dinosaur tree where birds diverged [6] , [7] , a diversity of paravian theropods is now known to have had well-developed feathers on their legs and tails, as well as on their arms (for example, Archaeopteryx, Microraptor , Anchiornis and Eosinopteryx ) [4] , [5] , [7] , [8] . Fossils also show that feathers first evolved for non-flight functions [9] , [10] . Phylogenetic studies nest long-tailed birds ( Archaeopteryx and relatives) within Paraves [6] , [7] ; as fossil members of several non-avialan lineages had well-developed, asymmetric feathers (equated with flight) [4] , [5] , it is certain that birds were not the only theropod lineage to possess some degree of aerial ability. Just how paravians utilized their feathered wings and what this may mean for the evolution of gliding and flapping remains much debated [1] , [11] , [12] . In this paper, we report on a series of wind tunnel tests performed to examine the flight performance of one feathered paravian pivotal to this debate—the five-winged dromaeosaurid Microraptor from the Early Cretaceous Jehol Biota of northeastern China [4] . The first theropod described with feathers on its arms, legs and tail (five potential lifting surfaces), Microraptor , implies that forelimb-dominated bird flight passed through a 4- to 5-wing ‘tetrapteryx’ phase [13] and/or represents an important stage in Cretaceous paravian flight experimentation. Owing to its functional and phylogenetic significance, the wing configuration and flight ability of Microraptor has been much debated. Previous interpretations have included the following: static interpretation of fossils [14] , computer-based flight performance modelling of fossils [15] , analysis of free-flying models [16] and scale model wind tunnel experiments [17] . No consensus on likely wing configurations (thus degree of stability and glide performance) has been attained as reflected in a factor of six range of predicted lift-to-drag (L/D) ratios in previous work (that is, in Chatterjee and Templin [15] : 15; Alexander et al. [16] : 4.1; Koehl et al. [17] : 3). L/D is one fundamental measure of flight performance determining minimum glide angle and thus maximum flight range under steady conditions. Results of our wind tunnel tests show that Microraptor would have been most stable while gliding at high-lift coefficients and consequently degraded L/D ratios. Flight simulations demonstrate that this behaviour had adaptive advantages, as sustaining a high-lift coefficient at the expense of high drag was the most efficient strategy for gliding from, and between, low elevations. Our results also demonstrate that anatomically plausible changes in wing configuration and leg position would have made little difference to aerodynamic performance. Significant to the evolution of flight, we show that Microraptor did not require a sophisticated, ‘modern’ wing morphology to undertake effective glides, as the high lift coefficient regime is less dependent upon detail of wing morphology. This is congruent with the fossil record and also with the hypothesis that symmetric ‘flight’ feathers first evolved in dinosaurs for non-aerodynamic functions, later being adapted to form aerodynamically capable surfaces. Wind tunnel experiments Performing wind tunnel experiments on a full-scale, feathered, three-dimensional (3D) Microraptor model that has accurate geometries, joint morphologies and feather orientations ( Fig. 1a ), (based on known fossils, see Methods), we tested different speeds, angles of attack and morphologies that encompass different anatomically feasible leg positions ( Fig. 1a inset). We feathered our model based on plumage descriptions [18] , selecting extant bird feathers of comparable length, and only used reconstructions that had limb geometries holding the asymmetric feathers in aeroelastically stable orientations (relative to airflow), as is always the case in extant birds (that is, with the narrower vane on the side of the feather facing the oncoming flow) [2] . For this reason, one recent, widely cited reconstruction for Microraptor is incorrect [4] , as it has asymmetric feathers subject to flow in the ‘wrong’ direction. 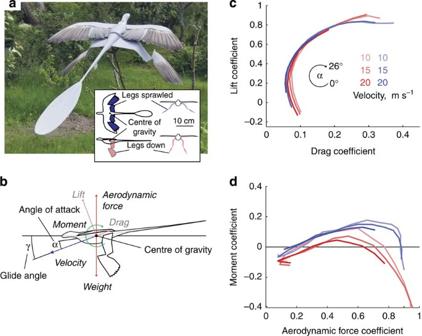Figure 1:Microraptormodel and measurement configurations. (a) Photograph of the full-scale feathered 3DMicroraptor(at Colin Palmer’s house on the Isle of Wight). Inset: main configurations. (b) Free-body diagram of a glidingMicroraptorshowing forces, moment and flight direction. (c) Measured lift and drag coefficients for the two main configurations. (d) Measured moment coefficient against aerodynamic force coefficient. Blue lines show results for the sprawled configuration, red lines legs down. The palest shades are at a wind tunnel wind speed of 10 m s−1, darkest 20 m s−1and intermediary shade 15 m s−1. In (c), the lines show the variation of lift and drag coefficients with increasing angle of attack (starting from bottom left at zero angle of attack). Force coefficients are the measured forces shown in the free-body diagram, nondimensionalized on the basis of projected area and dynamic pressure, the conventional approach used in aerodynamic analysis. In (d), the curves show the variation of the pitching moment coefficient and total aerodynamic force coefficient with increasing angle of attack (starting from the left at zero angle of attack). The pitching moment is a measure of the pitch stability. For stable flight, the gradient must be negative; therefore for these results, the models were only flight-stable at large values (>0.6) of total aerodynamic force coefficient. Figure 1: Microraptor model and measurement configurations. ( a ) Photograph of the full-scale feathered 3D Microraptor (at Colin Palmer’s house on the Isle of Wight). Inset: main configurations. ( b ) Free-body diagram of a gliding Microraptor showing forces, moment and flight direction. ( c ) Measured lift and drag coefficients for the two main configurations. ( d ) Measured moment coefficient against aerodynamic force coefficient. Blue lines show results for the sprawled configuration, red lines legs down. The palest shades are at a wind tunnel wind speed of 10 m s −1 , darkest 20 m s −1 and intermediary shade 15 m s −1 . In ( c ), the lines show the variation of lift and drag coefficients with increasing angle of attack (starting from bottom left at zero angle of attack). Force coefficients are the measured forces shown in the free-body diagram, nondimensionalized on the basis of projected area and dynamic pressure, the conventional approach used in aerodynamic analysis. In ( d ), the curves show the variation of the pitching moment coefficient and total aerodynamic force coefficient with increasing angle of attack (starting from the left at zero angle of attack). The pitching moment is a measure of the pitch stability. For stable flight, the gradient must be negative; therefore for these results, the models were only flight-stable at large values (>0.6) of total aerodynamic force coefficient. Full size image Wind tunnel model tests included two different leg configurations, two main wing angles of incidence relative to the body and two different tail sizes, all consistent with described Microraptor fossils and known microraptorine (dromaeosaurid) anatomy [4] , [19] . Tests also encompassed all previously proposed (anatomically feasible) wing configurations for Microraptor (Methods) ( Fig. 1a inset). Experiments were conducted for every configuration at three different flight velocities (covering a range consistent with those experienced by living gliding and flapping animals), from 10 to 20 m s −1 (refs 2 , 20 ) over an entire range of angles of attack ( Figs 2 , 3 , 4 ). An approximate location for Microraptor ’s centre of gravity (CoG) ( Fig. 1b ) was estimated based on reconstructions of described Chinese fossils [4] , [18] . This CoG location, which was used to determine pitching moment coefficients, was predicted to be 0.1 m behind the leading edge of the main wing ( Fig. 1b ). 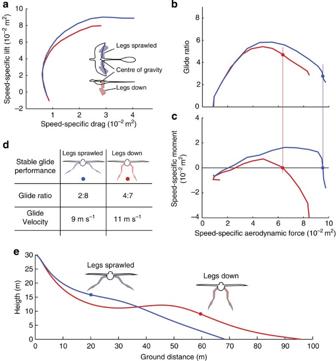Figure 2: Velocity-averaged aerodynamic performance of sprawled and legs down configurations. The forces are divided by the square of wind tunnel airspeed, thus allowing more direct comparisons between configurations of different projected areas than would be the case for conventional non-dimensional lift and drag coefficients. (a) Speed-specific Lift-Drag polar. It is apparent from this graph that the sprawled configuration (blue) produces more lift than legs down (red), a result obscured inFig. 1c. (b) Glide ratio against speed-specific aerodynamic force coefficient. The glide ratio is the ratio of lift:drag and is a measure of the glide angle. The higher the glide ratio, the shallower the glide angle. (c) Speed-specific moment coefficient against speed-specific force coefficient. Stable flight points occur where the pitching moment curve gradients are negative and the moment is zero. The graphs (b) and (c) share a commonxaxis; therefore, the stable flight points have been projected from (c) to (b) to determine the corresponding glide ratios. Although the sprawled configurations are capable of producing a higher glide ratio than legs down, the stability limit means that legs down actually achieves stable flight at a higher glide ratio. (d) Glide velocities and glide performance for the stable points. (e) Glide trajectories for the points in the stable regime. The curves show calculated flight paths for animals leaping from an elevated perch, flying at the aerodynamic conditions taken from the stable flight points. The legs down configuration initially falls further in order to build up a greater steady flight speed; therefore, for flights from heights of <15 m the sprawled configuration has the greater range. From heights of 2 m or more, legs down gives the greater range. Figure 2: Velocity-averaged aerodynamic performance of sprawled and legs down configurations. The forces are divided by the square of wind tunnel airspeed, thus allowing more direct comparisons between configurations of different projected areas than would be the case for conventional non-dimensional lift and drag coefficients. ( a ) Speed-specific Lift-Drag polar. It is apparent from this graph that the sprawled configuration (blue) produces more lift than legs down (red), a result obscured in Fig. 1c . ( b ) Glide ratio against speed-specific aerodynamic force coefficient. The glide ratio is the ratio of lift:drag and is a measure of the glide angle. The higher the glide ratio, the shallower the glide angle. ( c ) Speed-specific moment coefficient against speed-specific force coefficient. Stable flight points occur where the pitching moment curve gradients are negative and the moment is zero. The graphs ( b ) and ( c ) share a common x axis; therefore, the stable flight points have been projected from ( c ) to ( b ) to determine the corresponding glide ratios. Although the sprawled configurations are capable of producing a higher glide ratio than legs down, the stability limit means that legs down actually achieves stable flight at a higher glide ratio. ( d ) Glide velocities and glide performance for the stable points. ( e ) Glide trajectories for the points in the stable regime. The curves show calculated flight paths for animals leaping from an elevated perch, flying at the aerodynamic conditions taken from the stable flight points. The legs down configuration initially falls further in order to build up a greater steady flight speed; therefore, for flights from heights of <15 m the sprawled configuration has the greater range. From heights of 2 m or more, legs down gives the greater range. 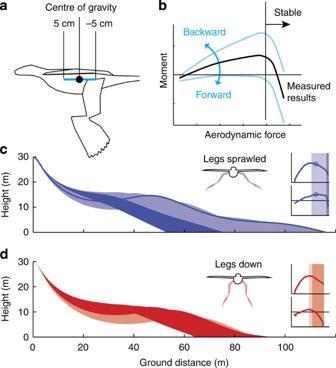Figure 3: Trajectory envelopes. The results inFig. 2are for one specific centre of gravity location; therefore, the effect of small variations in location were examined. (a) Range of centres of gravity considered. (b) Effect of changing the centre of gravity. Changing the location of the centre of gravity changes the shape of the pitching moment curves. (c) Trajectory envelope for legs sprawled. Dark-shaded area indicates stable glide. Dark line shows the best-performing glide trajectory, indicated by the point in inset. (d) Trajectory envelope for legs down. Dark-shaded area indicates stable glide. Full size image Figure 3: Trajectory envelopes. The results in Fig. 2 are for one specific centre of gravity location; therefore, the effect of small variations in location were examined. ( a ) Range of centres of gravity considered. ( b ) Effect of changing the centre of gravity. Changing the location of the centre of gravity changes the shape of the pitching moment curves. ( c ) Trajectory envelope for legs sprawled. Dark-shaded area indicates stable glide. Dark line shows the best-performing glide trajectory, indicated by the point in inset. ( d ) Trajectory envelope for legs down. Dark-shaded area indicates stable glide. 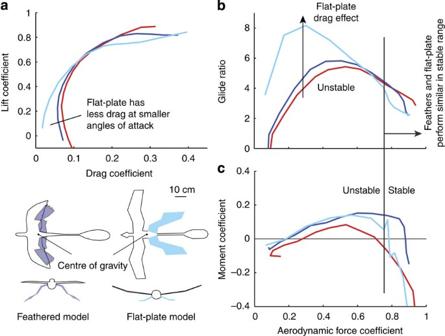Figure 4: Velocity-averaged aerodynamic performance in feathered and flat-plateMicroraptormodels. Results are shown for the sprawled configuration for feathered (dark blue lines) and flat (pale blue lines) plateMicroraptormodels. Results for the legs down configuration are shown in red for completeness. (a) Lift-Drag polar. (b) Glide ratio against aerodynamic force coefficient. (c) Moment coefficient against aerodynamic force coefficient. Full size image Figure 4: Velocity-averaged aerodynamic performance in feathered and flat-plate Microraptor models. Results are shown for the sprawled configuration for feathered (dark blue lines) and flat (pale blue lines) plate Microraptor models. Results for the legs down configuration are shown in red for completeness. ( a ) Lift-Drag polar. ( b ) Glide ratio against aerodynamic force coefficient. ( c ) Moment coefficient against aerodynamic force coefficient. Full size image Calculations We calculated L/D polars for Microraptor in different configurations ( Fig. 1c ) and plotted pitching moment coefficient against aerodynamic force coefficient ( Fig. 1d ). Although we tested three different configurations ( Fig. 1a inset), the force and moment coefficients we recovered do not vary greatly between configurations, and our moment coefficient curves ( Fig. 1d ) have similar shapes to the only previous model-based experimental study of Microraptor [17] . Results show that Microraptor could have changed its wing area by moving its legs into different positions and thus enlarging its force envelope ( Fig. 2a ). These differences in lifting wing surface area were taken into account using speed-specific L and -D (see Methods) [21] . Results also show that Microraptor would have aerodynamically (expressed by the glide ratio) performed best with the sprawled-leg configuration for all values of speed-specific aerodynamic force coefficient (SCR) ( Fig. 2b ). For stable points (lines connecting Fig. 2b,c ; see Methods for this calculation), the legs-down configuration has the higher aerodynamic efficiency (glide ratio 4.7 (:1)) compared with the sprawled-legs configuration (glide ratio 2.8 (:1)). Equilibrium glide velocities were calculated from the corresponding SCR with an estimated Microraptor mass of 0.5 kg (consistent with previous work) [15] , [16] , [17] , [22] ; this shows that lesser aerodynamic performance goes hand-in-hand with a lower glide velocity ( Fig. 2d ). Tests with different main wing angles and different tail areas show that a higher angle for the main wing (relative to the body and tail) decreases performance for stable glide conditions, and a change in tail area has no significant effect on aerodynamic performance or moment characteristics (see Methods). Taking the glide ratio and aerodynamic force coefficients for the two stable conditions identified ( Fig. 2d ), we then calculated flight trajectories solving for equations of motion ( Fig. 2e ; see Methods). Trajectories show that the most efficient glide trajectory requires a balance between aerodynamic efficiency and aerodynamic force. When leaping from a height of 30 m, the sprawled-leg configuration shows an initially shallower glide path; however, it ultimately falls short of the distance covered by the anatomically more likely legs down configuration [18] , [23] , which reaches 40% farther. Microraptor had the ability to flex and extend its forelimbs to bring the centres of aerodynamic force and CoG into coincidence, moving the balance point backwards or forwards ( Fig. 3a,b ). For a range of possible locations of the CoG, L/D–SCR combinations were used to create a trajectory envelope ( Fig. 3c,d ). For stable combinations, the sprawled-legs configuration is most effective in the early glide stage (<40 m) but cannot be used to glide as far ( Fig. 3c ). The legs-down configuration shows a balance between height loss in the early glide stage and the total distance travelled ( Fig. 3d ). When we take unstable balance points into account, the flight trajectories show that the sprawled-legs configuration could outperform the legs-down configuration ( Fig. 3c ). This means that Microraptor could fly even farther, if it had possessed an advanced flight-control system to maintain stable flight. However, it is unlikely that early flyers would have specialized and dedicated flight-control systems [24] , [25] . Results show that, irrespective of its wing configuration, Microraptor was aerodynamically unstable at low SCR ( Fig. 2c ) and would have been unable to glide with maximum aerodynamic efficiency (that is, high L/D). Thus, Microraptor would have been better off adopting a high SCR, lower L/D wing configuration to quickly generate the high lift at low speeds needed to minimize initial height loss in short glides from moderate heights. This high-lift, high-drag flight strategy ( Fig. 3 ) would have been very efficient for leaping from moderate heights ( ca. 20–30 m), consistent with tree sizes in the Jehol podocarp forest. Unsteady trajectory performance, rather than aerodynamic efficiency, seems to have been the main selective pressure optimised by Microraptor ’s flight style. Although comparative data from living birds [26] show that (if our fossil-based calculations are correct) the wing loading ( ca. 50 N m −2 ) of Microraptor is almost exactly at the mean for birds of the same weight, its L/D was much lower (many birds have L/D in the range 10–12 (ref. 26 ), whereas we calculate this for Microraptor at 4.7 (:1)). This must be, in part, because of the fact that (as we show) Microraptor ’s planform had an intrinsically less efficient configuration compared with living birds and also because it had to operate in a low-L/D region of its flight envelope in order to be aerodynamically stable. Even with legs deployed underneath the body and used to provide an initial push off, just a small horizontal velocity of up to 3 m s −1 would be generated [27] . This makes little difference to a flight path, as by far the bulk of necessary flight speed had to come from falling under the effect of gravity. As our experiments show that achieving a high SCR was most important for Microraptor ’s flight and that differences in gliding-leg position only lead to very small differences in performance, sprawled or legs-down configurations are equally likely, especially for medium-length gliding flights. Of these, however, a legs-down gliding configuration is best supported by fossil data [19] , [23] and has been shown to be advantageous in stabilizing roll and yaw [28] . Finally, in order to examine the effect of size as well as the necessity of feathers, we carried out further wind tunnel experiments comparing the feathered model in legs-sprawled configuration and in a matching but unfeathered model (Methods). Results demonstrate that Microraptor did not require well-developed flight surfaces to support its high C R (close to stall) flight style (that is, this flight capability was not very sensitive to airfoil section) ( Fig. 4 ). Flat-plate experiments show that in the region of sustained stable flight (that is, regions of high C R ; Fig. 4 ), there is very little difference in L/D between feathered and unfeathered models. The most important factor for this theropod was attaining sufficient wing area (for which derived feathers are unnecessary) to glide most effectively; theoretically, all Microraptor needed in order to glide at high C R would was an impervious surface. Our experimental results are, therefore, both congruent with, and build on, fossil evidence, showing that theropod filamentous integument and symmetric wing feathers first evolved for behaviours other than lift generation [9] , [10] . As our unfeathered model performs almost as well as our feathered one, results are congruent with the argument that gliding behaviours could have evolved in taxa with symmetric leg feathers (for example, Pedopenna [29] and Anchiornis [5] ). This further highlights the likelihood that asymmetric vanes were a further specialization that evolved in paravian taxa with gliding ancestors; in essence, these allowed a larger wing area for a given skeletal mass and removed the need for feather overlap. The gliding flight of Microraptor , which our experimental results show was remarkably effective over medium distances starting from moderate heights, did not require highly derived lifting surfaces and can be regarded as representing a highly successful experiment in theropod adaptation to aerial behaviour, consistent with at least some evidence for climbing in this taxon [30] . Providing a further comparative context for Microraptor ’s flight mode is complex because other four- and five-winged feathered dinosaurs possessed similar body plans. Clearly, Microraptor also lacks close analogues in the extant fauna, and its relatively high drag and potential unsteady trajectory imply that it might have combined arboreal and terrestrial foraging with rare, perhaps opportunistic, gliding behaviour (consistent with reports of fish in stomach contents [31] ). There are no strong indications from its aerial performance that it might have behaved similar to extant gliding mammals nor does it seems to have approached any extant volant birds in aerial performance. In sum, Microraptor likely indulged in some climbing behaviour, some terrestrial foraging behaviour and glided on occasion; it may thus have foraged across a vertical gradient, using a body plan different from that of extant species. The likely presence of microraptorines in the Late Cretaceous [19] combined with new evidence that a phylogenetically diverse range of Mesozoic birds [32] , including Archaeopteryx [8] , possessed feathered legs as well as wings suggests that this generalized, perhaps primitive, form of aerial adaptation was persistent across paravian history and was not a short-lived evolutionary event. Previous wing and flight reconstructions Several previous studies have considered the likely wing configuration(s) and flight performance of Microraptor ( Fig. 5 ). 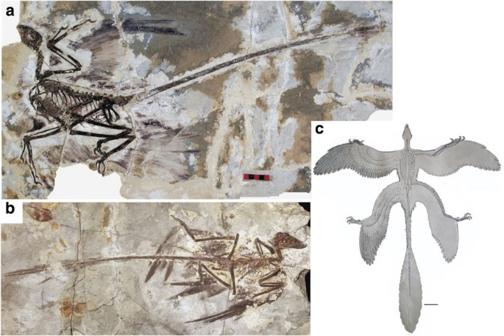Figure 5:Microraptorfossil specimens used as the basis for model making. Primary sources: (a) holotype specimen (Institute of Vertebrate Palaeontology and Palaeoanthropology, Institute of Vertebrate Palaeontology and Palaeoanthropology V13352) ofMicroraptor gui, and (b) fossil specimen (Beijing Museum of Natural History, BMNHC PH881) referred toMicroraptorby Liet al.18. Reference also made to (c), incorrect (see Methods) reconstruction of feathering. Figure 5: Microraptor fossil specimens used as the basis for model making. Primary sources: ( a ) holotype specimen (Institute of Vertebrate Palaeontology and Palaeoanthropology, Institute of Vertebrate Palaeontology and Palaeoanthropology V13352) of Microraptor gui , and ( b ) fossil specimen (Beijing Museum of Natural History, BMNHC PH881) referred to Microraptor by Li et al. [18] . Reference also made to ( c ), incorrect (see Methods) reconstruction of feathering. Full size image Chatterjee and Templin [15] reported results of a computer simulation of a gliding Microraptor using a biplane wing configuration, which they considered to be most anatomically plausible. On the basis of classical aerodynamic theory, they also expected this biplane configuration to be more efficient than tandem wings. Virtual models used for this work were based on measurements of fossil casts and digital reconstructions of wing planform. Chatterjee and Templin [15] analysed flight performance using two pieces of stream tube theory software [33] : ANFLTPWR (animal flight power) and ANFLTSIM (animal flight simulation) [33] (we have been unable, despite repeated attempts, to obtain copies of these codes from Chatterjee & Templin [15] , or to replicate their methods) and, in contrast to subsequent modelling work [16] , assumed that because of the biplane configuration the feathers on the femur and tibia only served to streamline and thus reduce the arodynamic drag of these leg bones and did not contribute to the production of lift. This study [15] concluded that likely flight speeds for Microraptor would have been between 9 and 15 m s −1 and that the dinosaur would have been a moderate glider, traveling from tree to tree in a phugoid motion, achieving at least 40 m of horizontal distance with a terminal flight speed of ca. 4.5 m s −1 , deemed to be safe for landing. Such estimates are highly dependent on the assumed L/D; therefore, if the much lower values reported by other workers were applied, the range would be greatly reduced. Alexander et al. [16] subsequently studied the aerodynamic properties of several different Microraptor configurations by producing free-flying models with wing profiles based on those of a pigeon. They based the overall shape on the Microraptor gui holotype (Institute of Vertebrate Paleontology and Paleoanthropology, Beijing) V13352 and investigated the following three configurations they considered plausible: the forewing and tail attached in the same frontal plane with varying incidence; the hind wings mounted with 20° of anhedral and 75° of sweep (similar to the previous configuration but with the tips of the hind wings horizontal); and a biplane configuration where the feet forming the hind wings are located beneath the main wing—a configuration supported by the earlier geometric study of Chatterjee and Templin [15] . Alexander et al. [16] tested their models as free-flying gliders and concluded that the mean steady-state glide ratio for each of their three configurations was 4.1 (ref. 16 ). The results, although showing much lower L/D ratio than theoretical predictions [15] , do indicate that gliding was feasible for Microraptor . Serious anatomical issues with the Microraptor model described by Alexander et al. [16] have, however, been raised: based on the known 3D anatomy of closely related microraptorines [19] , it is unlikely that Microraptor could have attained the leg positions used for this model [23] . Most recently, Koehl et al. [17] presented results of an experimental aerodynamic investigation of Microraptor using small physical models in a wind tunnel. Koehl et al. [17] used models based on Xu et al. [4] and compared the flight performance of Microraptor with its hind wings sprawled; laid flush along the tail; down; and in a biplane configuration. Wings were initially modelled with feathers; however, this was considered impractical, so most of the tests were conducted on models that had wings made from stiffened paper. Their results are similar to those reported by both Chatterjee and Templin [15] and Alexander et al. [16] , althought they were alone in providing limited results of the pitching moments and thus static pitch stability. Koehl et al. [17] went further to compare their results to modern bird-flight speeds, noting that estimated gliding speeds for Microraptor do fall within the range measured for extant taxa [34] . They also noted that there was no significant difference between the L/D ratios of the configurations that they reported; therefore, they concluded that the hindlimb position does not noticeably affect glide characteristics. Unlike earlier studies, Koehl et al. [17] discussed (but did not quantify) the effects of the position of the legs and their effect on glide stability, as well as the animals’ manoeuvrability and turning capabilities. Our model Microraptor was tested with all previously proposed leg configurations [15] , [16] , [17] , apart from the anatomically impossible, fully sprawled position [16] , as this would have been anatomically impossible [19] , [23] . Notes on Microraptor in a stable equilibrium glide For an animal gliding at velocity V, the only forces acting upon the body are the total aerodynamic force R, acting at the centre of pressure, and the weight of the animal W, acting at the CoG ( Fig. 6 ). Translating the total aerodynamic force to the CoG results in a moment M around the CoG. The animal can change these by (re)-arranging its lifting surfaces and/or by changing its (geometric) angle to the flow α . Furthermore, total aerodynamic force can be split into two components: one that is perpendicular to the flight direction, the lift L, and one that is in the opposite direction of flight, the drag D. The glide angle γ and glide ratio L/D are measures of glide performance. The higher the glide ratio (or the lower the glide angle), the higher the glide performance. 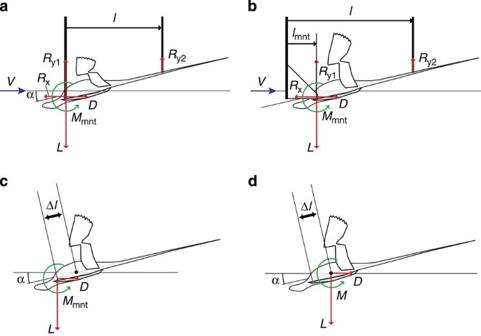Figure 6: Wind tunnel-mounting geometry of the modelMicroraptor. (a) Mounting for the sprawled configuration. (b) Mounting for the legs down configuration. (c) Moment and forces as measured. (d) Moment and forces around CoG.V=wind speed,α=angle of attack relative to the flow direction,L=lift force,D=drag force,Mmnt=pitching moment around mounting point,Rx=horizontal force measured by the force balance,Ry1andRy2=vertical forces measured at the attachment points.l=distance between attachment points andlmnt=attachment offset legs down. Δl=distance between mounting point and CoG.M=pitching moment around CoG. Figure 6: Wind tunnel-mounting geometry of the model Microraptor . ( a ) Mounting for the sprawled configuration. ( b ) Mounting for the legs down configuration. ( c ) Moment and forces as measured. ( d ) Moment and forces around CoG. V= wind speed, α =angle of attack relative to the flow direction, L =lift force, D =drag force, M mnt =pitching moment around mounting point, R x =horizontal force measured by the force balance, R y1 and R y2 =vertical forces measured at the attachment points. l =distance between attachment points and l mnt =attachment offset legs down. Δ l =distance between mounting point and CoG. M =pitching moment around CoG. Full size image For equilibrium glide, the total aerodynamic force and weight need to be equal in magnitude, in opposite directions, and collinear [35] . This means that the forces act at the CoG and the moment around it needs to be equal to zero. For a passive stable glide, the first requirement is static stability—that is, the stability derivative ∂ M /∂ α is smaller than zero over a finite range in α [35] . In most cases, this is equivalent to ∂ M /∂ R <0 over a finite range in R, as the total aerodynamic forces tend to increase with the angle of attack. The second requirement is dynamic stability; however, moderate active control of the lifting surfaces can easily counter any dynamic instability and is, therefore, of less importance. In short, for a passively stable equilibrium glide, the following three conditions must hold: This last criterion is generally equivalent to: Active stable glide removes the need for the latter criterion. However, it comes at the cost of an advanced flight-control system, which requires a considerable amount of computing power. It is unlikely that early flyers would have specialized and dedicated flight-control systems [24] , [25] . Model making Our wind tunnel model ( Fig. 1a ) was rendered in composite materials using measurements and body proportions of the Microraptor specimens described by Xu et al. [4] and Li et al. [18] . These two specimens have been uncontroversially referred to the same taxon and differ from one another only in their relative skeletal proportions and wing outlines; the M. gui holotype [4] is ca. 1/3 larger ( Fig. 5 ). As the specimen described by Li et al. [18] has already been rendered in 3D [18] , our model Microraptor has the proportions and wing outline of this specimen but was scaled up to fit comfortably into the working section of the University of Southampton (Engineering and the Environment) 2.1 m × 1.5 m wind tunnel. Owing to the known size range of specimens referred to as Microraptor [4] , [18] , [23] , [36] , an animal with proportions corresponding to our model existed in the Early Cretaceous Jehol Biota. Femur articulation at the pelvis and achievable angles between the femur, tibia and tarsals are based on Xu et al. [4] , Li et al. [18] and, critically, the only currently known 3D-preserved pelvis of a microraptorine dromaeosaur, the Canadian Hesperonychus [19] . Wing and leg feathers on our model Microraptor are from extant salvaged (Isle of Wight, UK, 2012) Mallards Anas platyrhynchos (outboard primaries) and Common wood pigeons Columba palumbus (inboard section) ( Fig. 1a ): measurements of the feathers of Mesozoic birds and selected theropod dinosaurs show that the primaries of Microraptor correspond most closely in relative length and width to those of mallards [37] . The projected areas of the main lifting elements (main wing area and projected area of the legs) were of 0.1085, m 2 for sprawled and 0.0899, m 2 for legs down. The large tail had an area of 0.0170, m 2 and the small tail an area of 0.0067, m 2 . The mean aerodynamic chord of the main wing (used to determine the moment coefficient) is 0.11 m. The location of the CoG is estimated to be ~0.1 m behind the leading edge of the main wing ( Fig. 1 ). To assess the influence of size (Reynolds number) and the influence of feathers (wing flexibility), a flat-plate Microraptor model in a sprawled configuration was used for experiments. This unfeathered model was constructed with Balsa wood for the main body, 2-mm thick aluminium flat plates for all lifting surfaces and a 1.2-cm aluminium rod for the tail (see Fig. 4a for planform and front view). The dimensions of this model were based on the holotype specimen of Microraptor in Xu et al. [4] The projected main lifting elements had areas of 0.1367, m 2 , whereas the tail had an area of 0.0147, m 2 . The mean aerodynamic chord of the main wing (used to determine the moment coefficient) is 0.11 m. The location of the CoG is estimated to be ~0.15 m behind the leading edge of the main wing ( Fig. 4a ). Wind tunnel experiments and analysis To assess the glide performance of Microraptor , we conducted wind tunnel experiments using different configurations of our feathered model ( Fig. 1a ). The influence of size and feathers was tested by conducting wind tunnel experiments on a flat-plate model and comparing these to the feathered results ( Fig. 4 ). The wind tunnel measurements were performed in the University of Southampton 7 × 5 ft wind tunnel (2.1 m × 1.5 m cross-section). A large-scale facility similar to this is needed to test full-scale models without suffering from wind tunnel-blockage effects. The air density was 1.2 kg m −3 . Lift, drag and moment ( L , D and M meas ) were measured using a three-component overhead balance system with accuracy: ɛ L =8 mN; ɛ D =2 mN; ɛ M =1 mNm. Each measurement was averaged over 75 samples. For the feathered model configurations, three velocities, 10, 15 and 20 m s −1 , and a range of geometric angles of attack ( α ), 0° up to 26° in 2° increments and back to 0°, were considered. Combinations that would result in forces that could damage the model were avoided. For each velocity, correction values—for the presence of mounting struts—for each α were determined by linear interpolation of the measured tare values (no model in the tunnel) for α =0° and α =27° and subtracted from the raw force and moment data. The data from the up and down α sweep were averaged. To avoid interference between the mountings and the legs, two different mounting setups were used ( Fig. 6 ). On an overhead balance, force can only be safely increased in a downward direction and, therefore, models are mounted upside down. In keeping with the real orientation, the model in Fig. 6 is depicted upside; the mount for the legs sprawled configurations is shown in Fig. 6a and the mount for the legs down configurations is shown in Fig. 6b . The moment acting on the animal around the mounting point is and, therefore, the measured moment can be used directly or, if needed, corrected by a factor of ( l – l mnt )/ l =0.7433 (with l mnt =0.145 m and l =0.565 m) to obtain the moment around the mounting point. The moment around the CoG was determined by: where Δ l is the difference between the mount location and the location of CG as shown in Fig. 6c,d . For the flat-plate model, the velocities measured ranged from 10 up to 25 m s −1 in steps of 5 m s −1 . Geometric angle of attack was varied from 0° up to 18° in 2° increments and, to capture stall accurately, from 18° up to 23° in 1° increments. The mounting and the correction of the raw data were similar to the sprawled configuration of the feathered model. Wind tunnel results were nondimensionalized using: ρ is the air density; V is the air velocity; S is the (projected) surface area of main lifting elements (main wing and hind wing) for each configuration; and c is the mean chord (based on main wing). Speed-specific forces and moment are determined using: C R S ; C L S ; C D S ; and C M S . Velocity-averaged results ( Figs 2 , 3 , 4 ) are averaged per AoA for all available velocities. Influence of the main wing angle and tail size To investigate the influence of the main wing angle (with respect to the body and tail), the angle of the main wing was increased by ±5° and all velocities and geometric angles of attack were repeated. The main difference is in the stall behaviour of Microraptor , which are shown as lower speed-specific L values ( Fig. 7 ). As a result, the glide performance for higher SCR decreases ( Fig. 7b ). The stable region and balance points are not changed significantly ( Fig. 7c ). 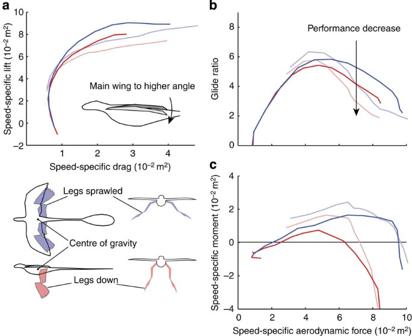Figure 7: Influence of the main wing angle on glide performance ofMicroraptor. The angle of main wing relative to the body (and tail) was varied by ~10 degrees. Dark lines: original wing position, blue sprawled, red legs down. Pale lines: wing at higher angle relative to body. (a) Speed-specific Lift-Drag polar. (b) Glide ratio against speed-specific aerodynamic force coefficient. The angled wings increase the best highest glide ratio but exhibit reduced values at higher aerodynamic forces. (c) Speed-specific moment coefficient against speed-specific aerodynamic force coefficient. Figure 7: Influence of the main wing angle on glide performance of Microraptor . The angle of main wing relative to the body (and tail) was varied by ~10 degrees. Dark lines: original wing position, blue sprawled, red legs down. Pale lines: wing at higher angle relative to body. ( a ) Speed-specific Lift-Drag polar. ( b ) Glide ratio against speed-specific aerodynamic force coefficient. The angled wings increase the best highest glide ratio but exhibit reduced values at higher aerodynamic forces. ( c ) Speed-specific moment coefficient against speed-specific aerodynamic force coefficient. Full size image The influence of tail size is investigated for configurations with the higher angle of the main wing ( Fig. 8 ) and, except for a few subtle changes in the moments around the CoG ( Fig. 8 ), no significant changes were found. 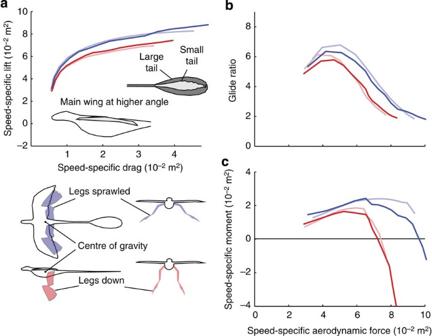Figure 8: Influence of tail size on glide performance ofMicroraptor. Colour coding as before. Bold lines: large tail (as used in all other tests), pale line:small tail. (a) Speed-specific Lift-Drag polar. (b) Glide ratio against speed-specific aerodynamic force coefficient. (c) Speed-specific moment coefficient against speed-specific aerodynamic force coefficient. Figure 8: Influence of tail size on glide performance of Microraptor. Colour coding as before. Bold lines: large tail (as used in all other tests), pale line:small tail. ( a ) Speed-specific Lift-Drag polar. ( b ) Glide ratio against speed-specific aerodynamic force coefficient. ( c ) Speed-specific moment coefficient against speed-specific aerodynamic force coefficient. Full size image Trajectory simulations Glide trajectories were determined by solving for the equations of motion in time to determine trajectories, using C L and C D combinations obtained from the measurements. Measurements of the gliding stage for real gliding animals [20] support that assuming constant C L and C D values are valid. The numerical approach is apparently similar to ANFLTSIM [15] , [33] , as far as we are able to replicate. At each time step, the equations of motion are solved: V is the total glide velocity; V d is the decent velocity; V h is the horizontal velocity; F x and F y are the forces in horizontal and vertical directions, respectively; a x and a y are the acceleration in horizontal and vertical directions, respectively; g is the gravitational acceleration; and m is the mass of the Microraptor . The velocity and location at the following time step are then determined by: where Δ t is the time step between successive evaluations; t is the time; and X and Y are the locations in horizontal and vertical directions, respectively. The mass of a Microraptor the size of our feathered model is estimated to be 0.5 kg. The start of the glide is at a height of 30 m, with an initial horizontal velocity of 3 m s −1 ( sensu Chatterjee and Templin [15] and in between experimental results for a European starling Sturnus vulgaris and Common quail Coturnix coturnix [27] ). Envelopes of glide trajectories were determined by finding the minimum and maximum heights of glide trajectories at each horizontal location. How to cite this article: Dyke, G. et al. Aerodynamic performance of the feathered dinosaur Microraptor and the evolution of feathered flight. Nat. Commun. 4:2489 doi: 10.1038/ncomms3489 (2013).